Single-particle structure determination by correlations of snapshot X-ray diffraction patterns Diffractive imaging with free-electron lasers allows structure determination from ensembles of weakly scattering identical nanoparticles. The ultra-short, ultra-bright X-ray pulses provide snapshots of the randomly oriented particles frozen in time, and terminate before the onset of structural damage. As signal strength diminishes for small particles, the synthesis of a three-dimensional diffraction volume requires simultaneous involvement of all data. Here we report the first application of a three-dimensional spatial frequency correlation analysis to carry out this synthesis from noisy single-particle femtosecond X-ray diffraction patterns of nearly identical samples in random and unknown orientations, collected at the Linac Coherent Light Source. Our demonstration uses unsupported test particles created via aerosol self-assembly, and composed of two polystyrene spheres of equal diameter. The correlation analysis avoids the need for orientation determination entirely. This method may be applied to the structural determination of biological macromolecules in solution. The advent of X-ray free-electron lasers (FELs) promises to eliminate the resolution limitation imposed on imaging of biological materials by radiation damage [1] . Owing to the extreme brevity and high fluence of the FEL pulses, even though a radiation dose at the target far exceeds the ‘safe dose’ radiation limit for conventional macromolecular crystallography [2] , diffraction is recorded before the onset of the structural damage processes [3] , [4] . In the single-shot diffraction serial nanocrystallography experiments at the Linac Coherent Light Source (LCLS), structure factors for lysozyme have been measured to 1.9 Å resolution [5] . Resolution in reconstructions of two-dimensional (2D) electron density projections for a large submicron virus [6] , soot and other aerosols [7] , [8] from single-shot LCLS diffraction patterns ranges from 24 to 41 nm. The next aim is experimental determination of three-dimensional (3D) structure from non-crystalline single particles using LCLS single-shot diffraction [3] . For most systems of practical interest, such as protein complexes, the experiment will be characterized by the small number of scattered photons, immersed in the high background noise, and uncertain number of particles in each shot. A weak signal dictates the necessity to use a complete data set of diffraction patterns from particles in random orientations to construct a 3D diffraction volume. The corresponding algorithms are based on expectation maximization (EM) [9] or dimensionality reduction [10] , [11] . They generally require each diffraction pattern to be generated by a single particle, posing practical constraints on the experiment. Instead of orientation classification of diffraction patterns, Kam proposed the simple averaging method that overcomes these constraints, and also reduces the vast data amount to a single compact 3D array. He demonstrated that averaging angular autocorrelation functions of individual 2D diffraction patterns yields the autocorrelation function of the 3D diffraction volume for a single particle, and this function can be related to the expansion coefficients of the diffraction volume in spherical harmonics [12] . Although Kam originally proposed his method for solution X-ray scattering, it has never been realized in this form owing to limitations of previously available X-ray sources. The most notable of these limitations arises from the restricted X-ray intensity from synchrotrons, such that statistically meaningful signal cannot be obtained during exposures shorter than the time for rotational diffusion on a length scale smaller than the desired resolution. Nevertheless, 2D projections of protein complexes immobilized on a supporting membrane have been successfully produced from correlations in cryo-electron microscopy images [13] . Recently, a correlation analysis was applied to soft X-ray imaging of 90-nm gold rods lying on the substrate perpendicular to the direction of X-rays, with many identical particles per shot [14] . Angular cross-correlation function for the speckle diffraction pattern has been used to reveal hidden local symmetries in colloidal systems [15] . With ultra-short and intense X-ray pulses from FELs, the requirement of the sample being frozen in time is easily satisfied in solutions at room temperature or in vacuum even for the smallest proteins, opening a door for measurements of spatial frequency correlations. Here, we report the first experimental demonstration of Kam’s method for particles with cylindrical symmetry arbitrarily oriented in space, that became possible with FELs. We utilized the LCLS to collect a set of single-shot diffraction patterns from unsupported known objects in random orientations. Owing to cylindrical symmetry the orientation is determined by two rotational degrees of freedom, and the particle shape is fully defined by the cross-section through the rotational symmetry axis. From the correlation analysis of the collected diffraction patterns, we obtained the diffraction volume of the oriented single particle and reconstructed its shape using a phase retrieval algorithm. This demonstration provides an experimental foundation of Kam’s method to diffractive imaging with X-ray FELs, and shows its potential for imaging biological macromolecules. Characterization of experimental diffraction patterns The test particles, considered in this work, consist of two touching polystyrene spheres (mean diameter of 91 nm), henceforth referred as sphere dimers. A set of 635 diffraction patterns from single particles with random orientation distribution was selected for analysis. 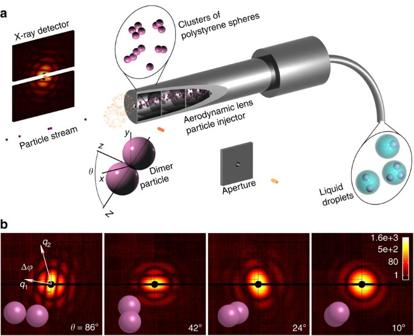Figure 1: Measuring single-shot diffraction patterns. (a) Experimental schematic. Micron-sized droplets emitted from an atmospheric pressure nebulizer contain one or multiple polystyrene spheres. As the droplets transit into the aerodynamic lens stack in a N2carrier gas, evaporation leads to single spheres or aerosol-assembled aggregates of random configurations. These particles accelerate towards the interaction region with a velocity of about 150 m s−1. LCLS X-ray pulses scatter off randomly intersected particles to produce a diffraction pattern recorded on the pnCCD. The unperturbed X-ray beam passes through a hole in the detector. Non-intercepted particles are captured in a particle beam dump. (b) Experimental diffraction patterns from dimers in several orientations, as indicated in the bottom of each image. The incident X-ray fluence, from left to right, is (3.7, 2.9, 4.4, 4.0) × 1010photons μm−2. Colourbar indicates detector counts. Detector gain is 7 counts per photon, and quantum efficiency is 0.9. Projections of the particles on the plane perpendicular to the X-ray beam direction, corresponding to each shot are also shown. Figure 1 shows a schematic of the experimental set up, and a representative set of diffraction patterns from dimers in various orientations, with corresponding particle projections as seen by X-rays. The X-ray fluence in each shot was estimated by extrapolation of the radially averaged diffraction patterns to the scattering vector q =0 following the procedure given in the Supplementary Methods , and varied from 8.5 × 10 9 to 2.3 × 10 11 photons μm −2 . To compensate for these fluctuations, we used deviations of photon count I ( q ) from the spherically averaged scattered intensity S ( q ), normalized by S ( q ): . This normalization also facilitates reliable determination of non-vanishing singular values of partial correlation matrices discussed further. The normalization factor S ( q ) was obtained as the radial average of the sum of all diffraction patterns. Before normalization of each pattern it was scaled to match the corresponding X-ray fluence. A small constant background has been added to each diffraction pattern and scaled S ( q ) to minimize a relative error in background subtraction for different shots. Figure 1: Measuring single-shot diffraction patterns. ( a ) Experimental schematic. Micron-sized droplets emitted from an atmospheric pressure nebulizer contain one or multiple polystyrene spheres. As the droplets transit into the aerodynamic lens stack in a N 2 carrier gas, evaporation leads to single spheres or aerosol-assembled aggregates of random configurations. These particles accelerate towards the interaction region with a velocity of about 150 m s −1 . LCLS X-ray pulses scatter off randomly intersected particles to produce a diffraction pattern recorded on the pnCCD. The unperturbed X-ray beam passes through a hole in the detector. Non-intercepted particles are captured in a particle beam dump. ( b ) Experimental diffraction patterns from dimers in several orientations, as indicated in the bottom of each image. The incident X-ray fluence, from left to right, is (3.7, 2.9, 4.4, 4.0) × 10 10 photons μm −2 . Colourbar indicates detector counts. Detector gain is 7 counts per photon, and quantum efficiency is 0.9. Projections of the particles on the plane perpendicular to the X-ray beam direction, corresponding to each shot are also shown. Full size image As a uniform distribution of particle orientations is essential for correct evaluation of correlation function, we estimated this distribution using the common-lines method [16] and cross-correlations with model diffraction patterns ( Supplementary Methods ). Though we found deviations from the uniform distribution, this did not significantly impact the results. Correlation analysis The arguments of the autocorrelation function for diffraction volume are the magnitudes of the two scattering vectors and the angle between them. After sampling each diffraction pattern corresponding to an unknown, random orientation ω in polar coordinates ( q n , ϕ m ), where n =1 ..N , m =1.. M , its angular autocorrelation function was computed as Averaging these functions over all diffraction patterns generates the autocorrelation function for a 3D diffraction volume C 2 ( q i , q j ,Δ ϕ k ). The magnitudes of scattering vectors q i and angles between them Δ ϕ k are calculated taking into account the curvature of the Ewald sphere, which resulted in the missing angles within 1.5° of Δ ϕ =0, and 3° in the vicinity of Δ ϕ =180°. Expansion of C 2 ( q i , q j ,Δ ϕ k ) as a function of angle in Legendre polynomials yields partial correlation matrices , where I lm is the column vector of normalized partial scattered intensities (expansion coefficients of scattered intensity in spherical harmonics, see Methods) with elements ( I lm ) i = I lm ( q i ) and is its adjoint. In general, these are N × N real symmetric matrices of at most rank 2 l +1, depending on the sample symmetry, which can be decomposed into the sum of rank-one matrices . While there are many ways to present a matrix as the sum of rank-one matrices, this can be most efficiently done by singular value decomposition (SVD, equivalent to eigenvalue decomposition for a hermitian matrix to within the signs of eigenvalues). It captures the maximum possible fraction of the matrix norm in the leading terms, corresponding to the largest singular values. That implies that if there are selection rules imposed on I lm by the particle symmetry, this will be reflected in the number of non-vanishing singular values for each l . Simplification of the analysis by a proper choice of the basis for the scattered intensity expansion based on the particle symmetry was demonstrated in the special case of icosahedral symmetry [17] . From SVD of the experimental partial correlation matrices, we found that all of them have rank one. That immediately implies the cylindrical symmetry of the diffraction volume, with the only contributions into its expansion coming from spherical harmonics with m =0. Corresponding partial scattered intensities I l 0 ( q ) can be calculated to within a sign as the product of the square root of the sole singular value and its singular vector. The signs of real partial scattered intensities still remain uncertain as so far we only used their products . They can be uncovered by involving spherical harmonics expansion of the squared scattered intensity I 2 ( q )/ S 2 ( q ) with coefficients Q l 0 ( q ), that has connection to the three-point autocorrelation function C 3 ( q i , q j ,Δ ϕ k ) computed at two scattering vectors from experimental diffraction patterns. General problem of unique determination of I lm ( q ) for the particles without symmetry using the higher-order correlation functions was addressed by Kam [18] . Similar to pair correlations, normalized partial triple correlations can be experimentally found and written in the matrix form as Like C 2 l , the matrix C 3 l is of maximum rank 2 l +1 and real. However, it is asymmetric as follows from equation 2. Limiting our discussion to an object with cylindrical symmetry, vectors can be calculated using equation 2: where ||·|| is a vector 2-norm. The same vectors can be also computed directly from pair correlations as quadratic forms of partial scattered intensities (Methods). Vectors and will coincide if all I l 0 have proper signs. Therefore, the signs can be determined by minimization of the difference between these vectors, defined by the R -factor , using signs of I l 0 as fitting parameters. The R -factor for all sign combinations up to l max =26 is plotted in Fig. 2a . The sets of and vectors for the sign combination corresponding to the point with the smallest R -factor are compared in Fig. 2b . This point can be clearly identified and correctly determines signs of all partial intensities. Alternatively, we can search for the sign combination that minimizes the number of negative pixels in the scattered intensity assembled from its spherical harmonics expansion. However, this method only gave us correct signs up to l =22. 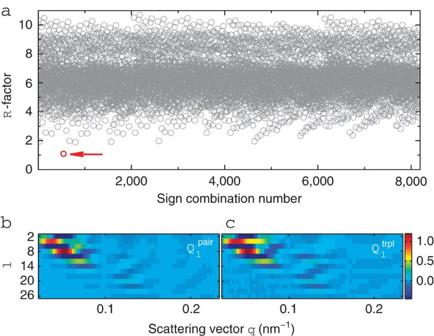Figure 2: Determining the signs of partial scattered intensities. (a)R-factor monitoring agreement between spherical harmonics expansion coefficients of the squared scattered intensity computed in two distinct ways for all possible sign combinations assigned to the first 13 non-vanishing partial scattered intensities withl>0. The arrow marks the point corresponding to the correct sign combination. (b,c) Comparison of the expansion coefficients of the squared scattered intensity calculated from pair and triple correlations, respectively. Each row corresponds to the differentl, indicated on the vertical axis, and magnitude is encoded with colour. Figure 2: Determining the signs of partial scattered intensities. ( a ) R -factor monitoring agreement between spherical harmonics expansion coefficients of the squared scattered intensity computed in two distinct ways for all possible sign combinations assigned to the first 13 non-vanishing partial scattered intensities with l >0. The arrow marks the point corresponding to the correct sign combination. ( b , c ) Comparison of the expansion coefficients of the squared scattered intensity calculated from pair and triple correlations, respectively. Each row corresponds to the different l , indicated on the vertical axis, and magnitude is encoded with colour. Full size image Partial scattered intensities I l 0 ( q ) S ( q ) up to l =26 with the signs correctly resolved from Fig. 2a are plotted in Fig. 3 by circles. They can be compared with the results of direct computation from the particle shape, described in Supplementary Methods , and plotted by solid lines. Now the determined partial scattered intensities can be substituted into the spherical harmonics expansion of scattered intensity to generate the diffraction volume. Owing to the cylindrical symmetry of the sample, the diffraction volume is fully defined by its azimuthal projection, which is equivalent to the central section through the axis of cylindrical symmetry. These sections, calculated directly from the model particle shape and experimentally determined partial scattered intensities, are depicted in Fig. 4a , respectively. The negative pixels in the experimental diffraction pattern were set to zero. 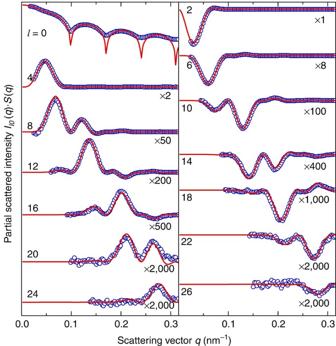Figure 3: Partial scattered intensities for the dumbbell-shaped particle. Circles correspond to computation from the experimental data. The result of calculation from the ideal particle shape is shown by solid lines. The degrees of spherical harmonics and scaling factors are indicated. Isotropic contributionl=0 is plotted in logarithmic scale. Figure 3: Partial scattered intensities for the dumbbell-shaped particle. Circles correspond to computation from the experimental data. The result of calculation from the ideal particle shape is shown by solid lines. The degrees of spherical harmonics and scaling factors are indicated. Isotropic contribution l =0 is plotted in logarithmic scale. 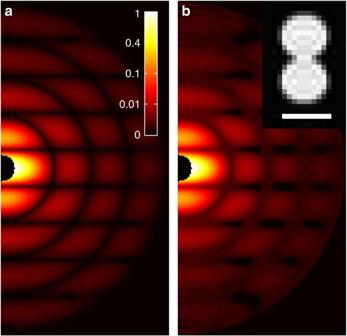Figure 4: Azimuthally averaged single-particle diffraction patterns. (a) Model partial scattered intensities (solid lines inFig. 3) are used for calculation of diffraction pattern. (b) Diffraction pattern is assembled from the experimental partial scattered intensities (circles inFig. 3) obtained by correlation analysis of randomly orientated diffraction patterns. Inset shows the image of azimuthally averaged electron density reconstructed from the experimental pattern. Scale bar is 10 nm. Full size image Figure 4: Azimuthally averaged single-particle diffraction patterns. ( a ) Model partial scattered intensities (solid lines in Fig. 3 ) are used for calculation of diffraction pattern. ( b ) Diffraction pattern is assembled from the experimental partial scattered intensities (circles in Fig. 3 ) obtained by correlation analysis of randomly orientated diffraction patterns. Inset shows the image of azimuthally averaged electron density reconstructed from the experimental pattern. Scale bar is 10 nm. Full size image Electron density reconstruction The diffraction pattern in Fig. 4b was used to solve the phase problem and reconstruct the sample electron density. In cylindrical coordinates, the azimuthal projections of the sample electron density and scattering amplitude are related by a Fourier transform in the direction of cylindrical symmetry axis and a zeroth-order Hankel transform in the radial direction [19] . While the 2D Fourier transform results in the projection of sample electron density in the direction of X-ray beam, this transform provides more information on the sample electron density by revealing the interior of the particle. For a sample with cylindrical symmetry, it is equivalent to a 3D Fourier transform of diffraction volume, and greatly reduces computation time. Image of the electron density averaged over 5,000 reconstructions with different starting points after their longitudinal alignment is shown in the inset of Fig. 4b . Full-period resolution is 20 nm, twice the pixel size, and limited by the maximum measured scattering vectors. The major sources of error in our analysis likely originate from the bias in the particles orientation distribution, mostly caused by the small size of the data set, and to some extent by the possible anisotropy introduced by the particle delivery system. Additional error can be introduced during the data selection and processing. Close resemblance between the single-sphere diffraction pattern and that of a dimer nearly aligned along the X-ray direction leads to the potential exclusion of such orientations from the analysis. Overrepresentation of the diffraction patterns, corresponding to the particles oriented perpendicular to the incident beam, may result from our data normalization by the incident X-ray fluence. As estimated in the Supplementary Methods , the fluence for such particles could be underestimated by as much as 25%. With an extensive data set, the normalization by X-ray fluence could be omitted if all classes of sample orientation are adequately represented over the entire distribution of observed X-ray fluences, and its fluctuations would be averaged out. We emphasize that although our test sample’s cylindrical symmetry has certainly simplified the correlation analysis, this symmetry was apparent from the form of the partial correlation matrices, each of which had a single singular value. Therefore, it did not need to be assumed a priori . The treatment of an arbitrary object lacking symmetries was given by Kam [20] . In this case, each partial scattered intensity I lm ( q ) is a linear combination of the 2 l +1 singular vectors of the corresponding correlation matrix. All I lm ( q ) for a given l can be found by multiplication of a special solution from SVD by a specific unitary matrix. Determination of these matrices for all l requires solving the optimization problem on the set of random unitary matrices (whose elements are additionally constrained by the properties of the spherical harmonics expansion coefficients) with the total number of parameters for expansion up to l max , which seems to be a formidable task. But many biological systems of interest are oligomers with some symmetry. In special cases, this symmetry will greatly decrease the number of fitting parameters. We expect that use of SVD will help to reveal the sample symmetries. As a simple example, the number of non-zero singular values for each l would identify the n -fold rotational symmetry. In a past similar experiment, a set of the soft X-ray diffraction patterns from ellipsoidal particles with variable X-ray fluence was converted into the 3D diffraction volume using the iterative expansion—expectation maximization—compression (EMC) algorithm [21] . EMC maximizes the log-likelihood function of the statistical model for the 3D diffraction volume parameterized by the scattered intensities on the Cartesian grid in reciprocal space. However, assembling the 3D diffraction intensities with the EMC requires each diffraction pattern to be produced by only a single particle. We avoid this restrictive requirement in our paper as single-particle correlation functions will be obtained even if more than one particle contributes to each diffraction pattern. Two factors permit this: first, averaging of the correlation function over all recorded diffraction patterns ‘washes out’ random cross-correlations and the coherent interference between different particles; second, for spatially separated particles, interference speckles are averaged out when the pixel size is adjusted to give a minimum oversampling required for reconstruction. The number of particles illuminated by X-rays in a single shot usually can be adjusted over a broad range if the sample is injected by means of aerodynamic lens stack [22] or liquid jet [23] . The ability to make productive use of multiple-particle diffraction patterns allows the significant sample dilution required to guarantee the predominance of single particle hits to be avoided. The allowed number of particles per shot is only limited by the detector intensity resolution or maximum sample concentration. Nevertheless, we should note that although computing correlations using a single diffraction pattern from N particles appears equivalent to averaging N correlation functions of single-particle diffraction patterns, the undesirable background is proportional to N 2 and N in the respective scenarios [18] . As demonstrated elsewhere [24] , the signal-to-noise ratio quickly saturates as the number of particles per shot increases. Besides the obvious advantages of reducing experimental time and computational load, in the multiple-particle diffraction, normalization by the radially averaged sum of all diffraction patterns can be replaced by normalizing each pattern by its radial average, as it approximates the spherical average of scattered intensity from the individual particle. That eliminates the requirement to determine the incident X-ray fluence in each shot. As the computation of correlations is simple and straightforward, it can be easily parallelized and even performed during experiments for useful and immediate feedback to experimenters. The resultant correlation functions are compact, when compared with the massive set of the original diffraction patterns, easy to manipulate and transfer between computers. It is instructive to note that the correlation functions in this paper can still be computed using measurements from detectors with sparse pixel distributions, as long as the entire required range of scattering vectors and their relative orientations is represented. In particular, the presence of the gap between the two detector halves in our experiment did not handicap the analysis. In summary, we have presented the first experimental evaluation of the use of the scattered intensity correlations to obtain and phase the single-particle diffraction pattern utilizing an ensemble of 2D snapshot diffraction patterns from nearly identical unsupported particles in random orientations, produced by an X-ray FEL. The size and electron density of these particles are similar to those of large viruses. Achievable resolution will be improved as harder X-rays with higher intensities are used, and stable submicrometre liquid jets for background minimization are developed. Our work highlights several important practical concerns in designing experiments aimed at structure determination through the use of spatial correlations. The many strengths of the spatial correlations approach discussed in this paper and its references continue to motivate and guide us in the ultimate goal of reconstructing the 3D structure of non-crystalline particles without symmetries. Data acquisition and sorting Experiments were carried out in the CFEL-ASG Multi-Purpose (CAMP) instrument [25] on the atomic, molecular and optical science (AMO) beamline at the LCLS. A colloidal suspension of polystyrene spheres (from Postnova Analytics GmbH), with nominal diameter of 98 nm, in water was atomized using a Mira Mist CE nebulizer (Burgener Research Inc., Mississauga, ON, Canada). Evaporation of water from the aerosolized droplets resulted in formation of self-assembled clusters of polystyrene spheres. They were focused and directed into the X-ray interaction region with help of a differentially pumped aerodynamic lens stack [22] , as illustrated in Fig. 1a . Clusters varying in size from a single sphere to large aggregates populate the particle beam. As we need to differentiate the dimer particles, the sample formation and delivery system was tuned to provide exactly one particle in each shot, similar to previous work [21] . Those particles that were intercepted by X-ray pulses produced diffraction patterns, captured by a detector system consisting of two 1024 × 512 pnCCD detectors located at the distance 738 mm from the interaction region, and separated by a gap of 1.6 mm. The pixel size was 75 × 75 μm 2 . This arrangement corresponds to full-period resolution of 20 nm for X-ray energy of 1.2 keV used in the experiment. The X-ray beam was focused to a 10 μm 2 focus spot in the interaction region. After removing the persistent background, faulted and saturated pixels, recorded diffraction patterns were preliminarily sorted by the total scattered intensity to eliminate empty shots and weak patterns. Images corresponding to sphere aggregates were extracted by selection based on the position of the first pronounced minimum in the radially averaged diffraction patterns. Patterns from single spheres were identified by flat angular autocorrelations. Finally, the set of diffraction patterns produced by dimers was selected by visual inspection of the remaining data. The average beam centre and relative position of two detector halves were determined by minimizing variations of the angular correlations in single-sphere diffraction patterns, or by maximizing the depth of minima in the radially averaged diffraction patterns. These two methods gave the same results. The set of 10,190 single spheres was used to determine the true size distribution of the spheres. For this purpose, the radially averaged scattered intensities were fitted to an analytical dependence using incident X-ray fluence, sphere radius and uniform background as fitting parameters. Owing to the small sphere size and low electron density of polystyrene, the phase shift introduced by a sphere is small, and scattered intensity can be calculated in the framework of the Rayleigh–Gans formalism [26] . The sphere diameter from this analysis is 91±5 nm (below the nominal size), which closely matches a simple estimation from the position of the first minimum in radial intensity. Variations in the determined sphere size also include apparent changes owing to the jitter in sample–detector distance of a few mm during the experiments, and possible effects of the X-ray pulse duration, intentionally varied from 70 to 300 fs. A total of 845 diffraction patterns from randomly oriented dimers were identified. Of these, the patterns whose first radial minimum was beyond the ensemble’s s.d. were excluded from examination in order to provide size monodispersity, a property essential for successful application of correlations. Correlation functions Here, we outline the relationships between the correlation functions and spherical harmonics expansions of corresponding values. The two-point (pair) correlation function normalized by the spherically averaged scattered intensity S ( q ) is where . The subscript ω denotes orientation of the particle, and averaging is performed over all possible orientations. Using the orthogonality of rotation matrices and the addition theorem for spherical harmonics, one can show [12] that this correlation function can be expanded in Legendre polynomials P l ( x ): where ϕ is the angle between q 1 and q 2 , and I lm ( q ) partial scattered intensities in spherical harmonics expansion of the normalized scattered intensity In this expansion , and only even l terms contribute into the sum owing to the (−1) l parity of spherical harmonics and symmetry of scattered intensity with respect to reflection about the origin (Friedel’s law). The expansion coefficients, or partial correlation matrices, of equation 5 are determined as: In a complete analogy with pair correlation function, normalized three-point (triple) correlation function calculated in two points is defined as Its evaluation requires expansion of the square of the normalized scattered intensity . Just like pair correlation function, C 3 ( q 1 , q 2 , ϕ ) can be reduced to a set of expansion coefficients in Legendre polynomials There is a connection between expansion coefficients I lm ( q ) and Q lm ( q ), which can be established by taking square of equation 6 and using the product rule for spherical harmonics: where C ( l 1 l 2 l ; m 1 m 2 m ) are Clebsch–Gordan coefficients. Phase retrieval To obtain phases of the scattering amplitudes, the relaxed averaged alternating reflections algorithm [27] , a variant of iterative projection phasing algorithms, was used. A quasi-discrete Hankel transform [28] was applied for numerical calculation. A starting point in reciprocal space was generated by assigning random phases to the experimental scattering amplitudes, which were set to the square root of the azimuthal projection of diffraction volume. The initial support mask was estimated from the sample autocorrelation. The support was updated as iterations proceeded following the Shrinkwrap algorithm [29] . This algorithm periodically modifies the object support, using the current estimate of the object’s electron density. In addition to the support constraint, reality and positivity constraints were applied in real space. In reciprocal space, the unmeasured scattering amplitudes in the central beamstop area and pixels with zero values were kept unconstrained. To estimate consistency between independent reconstructions, we calculated the phase retrieval transfer function PRTF( q )=|〈exp( iϕ q )〉|, where ϕ q are retrieved phases, and averaging is performed over all reconstructions. Resolution can be defined by the point where radially averaged PRTF drops below 1/ e . For our reconstruction, PRTF falls to 0.47 at the maximum value of measured scattering vector, and resolution is diffraction limited. How to cite this article: Starodub, D. et al. Single-particle structure determination by correlations of snapshot X-ray diffraction patterns. Nat. Commun. 3:1276 doi: 10.1038/ncomms2288 (2012).